Drug export and allosteric coupling in a multidrug transporter revealed by molecular simulations Multidrug resistance is a serious problem in current chemotherapy. The efflux system largely responsible for resistance in Escherichia coli contains the drug transporter, AcrB. The structures of AcrB were solved in 2002 as the symmetric homo-trimer, and then in 2006 as the asymmetric homo-trimer. The latter suggested a functionally rotating mechanism. Here, by molecular simulations of the AcrB porter domain, we uncovered allosteric coupling and the drug export mechanism in the AcrB trimer. Allosteric coupling stabilized the asymmetric structure with one drug molecule bound, which validated the modelling. Drug dissociation caused a conformational change and stabilized the symmetric structure, providing a unified view of the structures reported in 2002 and 2006. A dynamic study suggested that, among the three potential driving processes, only protonation of the drug-bound protomer can drive the functional rotation and simultaneously export the drug. Multidrug resistance during infection and cancer treatment is a serious problem [1] , [2] . It is often caused by the overexpression of efflux transporters that pump drugs out. In E. coli , among many such transporters, the tripartite efflux system, AcrB–AcrA–TolC, is largely responsible for resistance against many lipophilic antibiotics [3] , [4] , [5] , [6] , [7] , [8] , [9] . The tripartite system spans the inner and the outer membranes of the cell, effectively transporting drugs from the cell to the medium, bypassing the periplasm [10] , [11] : TolC is a generic outer membrane channel in which drugs can passively move [12] , AcrB, a member of resistance-nodulation-cell division transporters, is the inner membrane transporter that pumps drugs from the cell to the TolC channel driven by the proton-motive force [13] , [14] , [15] , [16] , and AcrA is an adaptor that links AcrB and TolC [11] , [17] . Thus, the active pump in this tripartite system is primarily realized by AcrB. Moreover, AcrB is currently one of the best-characterized transporters, making it an ideal target for simulation study. For AcrB, the high-resolution structure was first solved in 2002 [13] . The structure clarified that AcrB is a homo-trimer assembled in a triangular-prism shape and each protomer comprises three domains, trans-membrane (TM) domain, porter domain and TolC docking domain (see Fig. 1a ). The TM domain must be responsible for the proton transfer across the inner membrane harvesting the driving energy. The porter domain is made of four subdomains, PN1, PN2, PC1 and PC2, and is responsible for the drug binding. TolC docking domain has a funnel-like shape with a central channel that connects to TolC. Notably, the structure was solved in the crystal with the threefold crystallographic symmetry ( R 32 space group). Thus the asymmetric unit contained only one protomer, which enforced the reconstructed trimer structure being symmetric. It was not clear whether the perfect symmetry is the intrinsic property of the molecules or, to some extent, the artefact of the crystal packing. 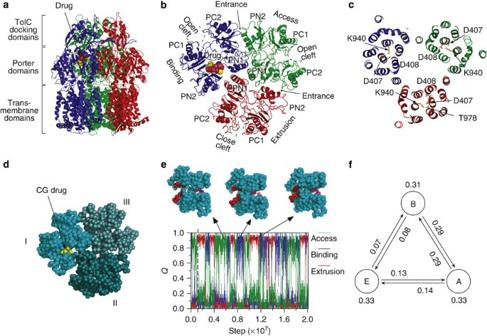Figure 1: The crystal structure and coarse-grained (CG) model of AcrB. (a) Side view of the crystal structure of AcrB; the drug molecule is represented by van der Waals' spheres. (b) Isolated porter domain viewed from the cell exterior. The protomers in blue, red and green represent the binding (abbreviated by B), extrusion (E) and access (A) states respectively. (c) Trans-membrane domain viewed from the cell exterior. The key residues around protonation sites are represented by sticks. (d) The CG model of the AcrB porter domain and the drug, minocycline (yellow). Two residues that hide the drug are not drawn. The chains being the B, E and A states in the crystal structure are numbered by I, II and III respectively. (e) A trajectory of conformational changes of the single protomer. The threeQscores (seeMethods) are plotted simultaneously, where the dashed line indicates the start for production. Representative snapshots for the three states are also shown above the time series, in which the red and pink spheres indicate key conformational difference. (f) Results for the single protomer simulation with the control set. The values near circles are the probabilities of corresponding states, whereas those beside arrows are transition frequencies between states. Figure 1: The crystal structure and coarse-grained (CG) model of AcrB. ( a ) Side view of the crystal structure of AcrB; the drug molecule is represented by van der Waals' spheres. ( b ) Isolated porter domain viewed from the cell exterior. The protomers in blue, red and green represent the binding (abbreviated by B), extrusion (E) and access (A) states respectively. ( c ) Trans-membrane domain viewed from the cell exterior. The key residues around protonation sites are represented by sticks. ( d ) The CG model of the AcrB porter domain and the drug, minocycline (yellow). Two residues that hide the drug are not drawn. The chains being the B, E and A states in the crystal structure are numbered by I, II and III respectively. ( e ) A trajectory of conformational changes of the single protomer. The three Q scores (see Methods ) are plotted simultaneously, where the dashed line indicates the start for production. Representative snapshots for the three states are also shown above the time series, in which the red and pink spheres indicate key conformational difference. ( f ) Results for the single protomer simulation with the control set. The values near circles are the probabilities of corresponding states, whereas those beside arrows are transition frequencies between states. Full size image This concern motivated crystallographers to solve the AcrB structure in a crystal that lacks the threefold symmetry, leading to the asymmetric trimer structures reported in 2006 and 2007 by three groups [14] , [15] , [16] . Interestingly, these new structures solved in different crystallographic symmetries were essentially identical to each other. In the new structure, albeit its overall similarity to the structure solved in 2002, the three protomers took somewhat different conformations, which may represent three particular stages during one functional cycle. Specifically, in the porter domain, one protomer (protomer I) took the 'binding' (denoted as B) conformation, where a drug molecule (for example, minocycline) was bound in a pocket formed by the three subdomains, PN1, PN2 and PC1 (blue chain in Fig. 1b ). Moreover, the B conformation has an evident open entrance, and thus is essentially the inward-facing state [18] . In the second protomer (protomer II), called 'extrusion' (E) conformation, one sees the exit path connected from the binding pocket to the central pore that is linked to the TolC channel, whereas the entrance gate is closed and the binding pocket is shrunk (red chain in Fig. 1b ). Thus, this is an outward-facing conformation. The third protomer (protomer III) took the 'access' (A) conformation, which resembles the B conformation except that the binding pocket is shrunk so that no drug molecule can be accommodated. This looks an inward-facing state to incorporate the drug (green chain in Fig. 1b ). The A conformation is very close to the structure solved in 2002 (C α root mean square deviation is 1.2 Å). The conformational difference among protomers is not only in the porter domain, but also in the TM domain which is crucial for the proton transport mechanism; D407 and/or D408 in the TM domain is likely to be protonated only in the E form, but not in the A or B form ( Fig. 1c ). The asymmetric structure of AcrB immediately led to the proposal of the functionally rotating mechanism [14] , [15] , [16] , by analogy to the binding change mechanism for ATP synthase [19] . Namely, starting from the BEA state (that is, the asymmetric crystal structure. Here, the first, second and third characters indicate the states of protomers in a counterclockwise order, for example, the protomers I, II and III respectively), after one functional step, the protomer I changes its state from B to E, the protomer II from E to A and the protomer III from A to B, in a coordinated way. As a trimer, this coordinated change results in the EAB state and thus can be viewed as the 120° rotation of the functional state when viewed from the outside. In three such steps, each protomer changes its state in a cyclic way, B→E→A→B, which may export one drug molecule per protomer. Although recent in vivo experiments indirectly supported this functionally rotating mechanism [20] , [21] , [22] , the difficulty in in vitro experiments precludes the more direct proof. Given this situation, molecular dynamics (MD) simulations may provide some further supports of the model, which is the purpose of this article. Although the MD simulations can be a powerful approach to provide high spatio-temporal resolution insights to transporter functions, the time scale reachable by the conventional all-atom MD is far below the time scale relevant to the AcrB functional cycle. Thus, some accelerations are often used, for example, the targeted-MD implemented in a recent study of AcrB, by which interesting drug translocation, but not the complete export, was observed [23] . Instead, here, we used a structure-based coarse-grained (CG) model recently developed based on the energy landscape perspective [24] , [25] , [26] , making much more comprehensive simulation possible. In particular, we represented each residue in the protein as a bead and used the multiple-basin model [25] , [27] , [28] . Here, using computational modelling, we address both the thermodynamics and the dynamics of the porter domain of AcrB. In the thermodynamics, one fundamental question is what caused the symmetry breaking. We investigated the relation between the symmetric structure solved in 2002 and the asymmetric one solved in 2006. In the dynamic study, we investigated the structural transition pathways: in a functional step from the BEA state, what is the order of conformational changes for protomers? In terms of energy, the first change is most likely driven by either the E→A (deprotonation) or the B→E (protonation). However, the detail is largely unknown and so we address this problem here. Modelling each protomer with the triple-basin CG model We start with the CG modelling of each AcrB protomer, for which the asymmetric AcrB structure suggests the presence of at least three stable states; the B, E and A states. The prerequisites to the AcrB trimer-complex simulations are to model the energy landscape that has the corresponding three basins and to realize simulations of conformational transitions between them. Given the crystal structures of the three states, we can easily achieve them by using the multiple-basin model [25] , [29] . The multiple-basin model was developed based on the energy landscape perspective of proteins [30] , [31] , [32] , [33] . The perspective clarified that proteins have evolved their sequences so that the overall energy landscapes resemble funnel-like shape enabling the proteins to fold to their native states sufficiently quickly. When magnified, the native basin often has multiple minima and transitions among them are crucial for their functioning. An ideal funnel-shaped landscape with only one native state can concisely be expressed by the topology-based model, called the Go model [24] , [34] . By smoothly connecting two or more Go models, the multiple-basin model realizes both the overall funnel-like shape towards the native basin and multiple minima within the native basin. This model has recently been applied to some biomolecular machines [25] , [27] , [28] . We used the multiple-basin model with triple basins corresponding to the B, E and A states of the AcrB protomer ( Supplementary Methods ). To the best of our knowledge, this is the first realization of the triple-basin energy landscape by structure-based methods. Here, only the porter domain of AcrB was considered and each amino acid in the protein was represented by a sphere centred at the C α atom ( Fig. 1d ). The drug was not explicitly treated in this and the next sections, but was included in the study of dynamics and drug export. In the triple-basin model of each protomer, there are two types of essential parameters that crucially affect the dynamics and the thermodynamics of the protein. The first parameter is the coupling constant Δ ij that controls the barrier height between the states i and j . For the two-basin case, the value of Δ can be inferred from experimental kinetic data [35] , if available. Here, however, without any prior knowledge we set all Δ ij equal (denoted as Δ). The change in Δ basically changes the time scale for all the transitions in the same way, but does not affect the thermodynamics or relative order of events. Thus, we set the value of Δ only for the computational reason; we used a sufficiently large absolute value of Δ so that transitions among the three states are realized within the allowed computer time (Too large absolute value of Δ is a problem, too. See Supplementary Methods ). The second type of parameters is the energy depths of the three basins, Δ V B , Δ V E and Δ V A , which controls the relative stabilities. One of the three parameters can be set as the reference (here Δ V A =0), so that the remaining two parameters (Δ V B and Δ V E ) are essential. For them, below we scanned broad range of values. As a preparation to the trimer-complex simulation described later, we sought a parameter set (Δ V B , Δ V E ) that results in the three states equally probable as a protomer, that is, the three states have the same free energy. By performing iterative MD simulations, we realized it with (Δ V B , Δ V E ) = (−8.6, −2.5) (in the energy unit of 4.17 k B T , where k B is the Boltzmann constant and T the simulation temperature). This will be used as the 'control' set, later. We note that the drug was not explicitly treated here and thus the low Δ V B value implicitly took into account some additional stability by the drug binding. A typical trajectory with this condition is illustrated in Figure 1e . The state of a protomer was quantitatively measured by the fraction of formation of certain native contacts (see Methods ). Figure 1e shows that the simulated protomer travels all the three states repeatedly in a single trajectory. The thermodynamics and the kinetics of the protomer in the 'control' set are summarized in Figure 1f . The populations of the three states (the numbers near the circles in Fig. 1f ) were indeed almost the same. Interestingly, the transition frequencies between the states (the numbers near the arrows) are not equal. The transitions between the A and the B states are the most frequent, whereas the transitions to and from the E state are somewhat slow. Especially the transition between B and E states is the slowest. By the choice of the equal coupling constant Δ, this reflects the difference in the distances between the conformations. The A and B conformations are relatively close, whereas the E state is somewhat far from the other two (see Supplementary Table S1 ). Allosteric coupling revealed by a thermodynamic study We now turn to the equilibrium thermodynamics of AcrB trimer where the allosteric coupling among the three protomers is crucial. To address the allostery, we need a careful computational modelling of the inter-protomer interface interactions, and so we took a multiscale approach. First, by the standard all-atom energy function, we estimated the inter-protomer interactions at each of the three interfaces, that is, the B/E, the E/A and the A/B interfaces, at the asymmetric BEA structure. Finding that strengths of contact energies depend on their conservation in the three interfaces, we classified the residue pairs at the interfaces into three sets (see Supplementary Methods ). The 'com3' set contains the residue pairs that make contacts in all three interfaces. These pairs have the strongest interactions. The pairs that make contact only at the two interfaces (called the 'com2' set) have the middle-strength interactions. The pairs that make contacts only at one interface are classified into the 'spec' set, which has the weakest interactions. For each set, based on the all-atom energy estimate, we assigned the CG contact strengths (see Methods and Supplementary Table S2 ). Combining these inter-protomer interactions with the intra-protomer model of the 'control' set (Δ V B , Δ V E )=(−8.6, −2.5) defined above, we simulated the AcrB trimer. The equilibrium ensemble thus obtained was dominated by the AAA state ( ∼ 60% in population), with some subdominant populations of the BBA and the AAB states ( Fig. 2b , the top left panel). This was understood by the analysis that, over the simulated ensemble, the inter-protomer average energies at the B/E, the A/E and the E/E interfaces are much weaker and thus unfavourable than other interfaces (see Supplementary Fig. S1 ). This is in harmony with the asymmetric crystal structure, where the B/E interface is markedly sparse and thus is weakly interacting ( Fig. 1b ). Moreover, the B/B interface interaction is also relatively weak. 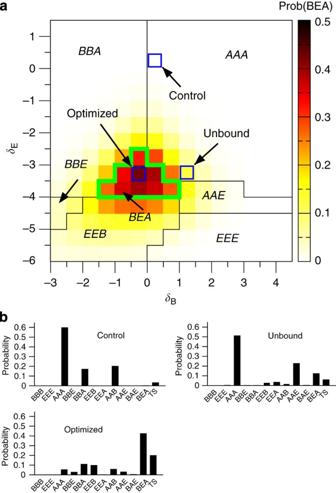Figure 2: Thermodynamics of the porter domain of AcrB. (a) Two-dimensional phase diagram. Thexandyaxes measure the variation of the stabilities of the B and E states respectively, with the 'control' as the reference (see text). Different phases are separated by solid lines, and the dominant configuration within each phase is indicated. The trimer configuration is represented by a triplet of characters, in which the first, second and third characters indicate the states of protomers in a counterclockwise order, e.g., the protomers I, II and III respectively. The phase where 'BEA' dominates is emphasized by the thicker green line. The three models used in this work, 'control', 'unbound' and 'optimized', are indicated by blue squares. The probability of 'BEA' on each point is expressed by colours. (b) Probabilities of all possible states for the three models. 'TS' means the transition state, in which one or more protomers stay in none of the three states. Figure 2: Thermodynamics of the porter domain of AcrB. ( a ) Two-dimensional phase diagram. The x and y axes measure the variation of the stabilities of the B and E states respectively, with the 'control' as the reference (see text). Different phases are separated by solid lines, and the dominant configuration within each phase is indicated. The trimer configuration is represented by a triplet of characters, in which the first, second and third characters indicate the states of protomers in a counterclockwise order, e.g., the protomers I, II and III respectively. The phase where 'BEA' dominates is emphasized by the thicker green line. The three models used in this work, 'control', 'unbound' and 'optimized', are indicated by blue squares. The probability of 'BEA' on each point is expressed by colours. ( b ) Probabilities of all possible states for the three models. 'TS' means the transition state, in which one or more protomers stay in none of the three states. Full size image Starting from the control set, we then altered the relative stabilities (Δ V B , Δ V E ) in the two dimensions, leading to the 'phase diagram' depicted in Figure 2a . Here, the 'phase' stands for the most probable trimeric state, which is not the rigorous 'phase' in classical thermodynamics. The boundaries between different phases are illustrated by lines. For the x and y axes, we used the deviation from the control, δ B =Δ V B −Δ V c,B and δ E =Δ V E −Δ V c,E respectively, where the subscript 'c' means the 'control'. The phase diagram was calculated by the standard histogram re-weighting method (see Supplementary Methods ). In the phase diagram ( Fig. 2a ), we found a triangular region in which the BEA state is dominant. Apparently, this corresponds to the asymmetric crystal structure. Thus, with the modelled allosteric coupling and a certain set of relative stabilities, the asymmetric structure can be a stable form, which validates the modelling. The population of the BEA was the largest at ( δ B , δ E )=(−0.5, −3.5) ( Fig. 2b , the bottom left panel), which was denoted as 'optimized'. We assume that this optimized value corresponds to the real BEA state as the asymmetric BEA state was found experimentally. Because the BEA state was found with one drug molecule bound to the B protomer, we now ask what would happen if the drug is dissociated. Computationally, the drug binding was effectively treated by a low Δ V B value, and so the drug dissociation corresponds to the increase in δ B . The phase diagram indicates that, by increasing δ B (moving to the right in the diagram), we almost surely reach the AAA phase where the AAA state dominates. Importantly, this AAA state is essentially the symmetric trimer structure obtained in 2002 because, as noted before, the A form is very close to the conformation in the structure solved in 2002. Although the drug binding energy is not accurately estimated here, we chose, only for illustration, ( δ B , δ E )=(1.0, −3.5) as a representative point for the drug unbound state (denoted as 'unbound'; see Fig. 2b , the top right panel, for the population). This leads to an important conclusion that, if the BEA structure is the stable structure with a drug bound to the B conformer, the drug dissociation most likely leads to the symmetric AAA structure. Figure 2a suggests that if we start from a non-optimal value of ( δ B , δ E ) in the BEA region, the dominant drug unbound state can be the AAE state. Even in this case, the probability of the AAA state is competitively high (see Supplementary Fig. S2 ). The conclusion here is also robust with respect to model parameters (see Supplementary Fig. S2 ). Functional rotation and drug export by the dynamic study Next, we studied the dynamic aspect of the AcrB function. Does the functional rotation really occur? Is the drug molecule transported to the outer membrane side? Addressing these questions, we performed a series of dynamic simulations of the drug export adding two more elements to the previous simulation system. First, we included one drug molecule explicitly represented by a CG model. Second, to form the natural 'exit' tunnel, we added a few more amino acids belonging to the TolC docking domain (see Methods ). More specifically, we set the initial state as the protomers I, II and III being in the B, E and A states, respectively. For the protomer I, the drug was explicitly included and thus the unbound δ B =1.0 was used, whereas for other protomers, we did not include the explicit drug and thus assumed the bound (optimized) δ B =−0.5. Assuming that the BEA state is one of the on-pathway functional states, we can think of three possibilities to go from the BEA state: the next event is activated either by the protomer I probably through protonation in the TM domain, by the protomer II probably through deprotonation in the TM domain or by the protomer III perhaps through the drug binding to the porter domain. We tested these three scenarios to address which is more likely. To mimic the activation by the deprotonation in the protomer II, during the simulation from the BEA state, we suddenly decreased the Δ V A value of the protomer II by 10.0 that induced the conformational change of this protomer to the A state (denoted as 'E→A' type). The same kind of switching was used to mimic the activation in the protomer I ('B→E') and the activation in the protomer III ('A→B'). For each case, after switching, we monitored what happened in the trimer state, as well as the drug originally bound in the protomer I. We start with the case of the activation in the protomer II (the E→A type). 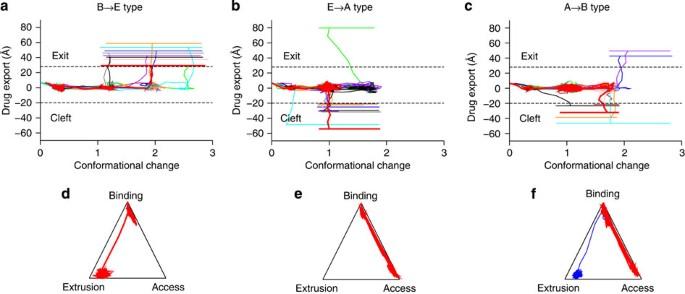Figure 3: Dynamic simulations for the functional rotation and the drug export of AcrB. Trajectories are distinguished by different colours, and the results of 'B→E', 'E→A' and 'A→B' type simulations (see text) are placed, in order, from the left to the right columns. In (a–c), dashed lines represent the criteria to determine whether the drug is exported through the 'exit' or 'cleft'. For clarity of the figures, once a trajectory goes across the thresholds, itsyaxis value is frozen whereasxaxis value continues to change. (d–f) Ternary plots of theQscores, which show the itinerancy of the state of protomer I (seeSupplementary Methods). Only representative trajectories are drawn for clarity. Figure 3b monitors the drug export (in y axis) and the conformational change (in x axis) for 10 independent trajectories. Here, the x axis indicates how many protomers completed their conformational changes; zero means the initial state and three means the complete transition to the EAB state. The y axis is a designed coordinate that reports the location of the drug (see Supplementary Methods and Supplementary Fig. S3 ); around zero at the binding pocket, the negative value (up to −20) along the 'cleft' tunnel (see also Fig. 1b ) towards the periplasm and the positive value (up to 28) towards the TolC-side exit. Thus the positive value indicates the functional drug export. In the current simulations, of the 10 cases, nine trajectories showed the drug export to the cleft direction (see also Supplementary Movie 1 ). On top, the conformational change did not complete for all 10 trajectories. The protomer I changed from the B to the A state in all cases ( Fig. 3e shows one example). All these consistently suggested that this is not the likely mechanism. Figure 3: Dynamic simulations for the functional rotation and the drug export of AcrB. Trajectories are distinguished by different colours, and the results of 'B→E', 'E→A' and 'A→B' type simulations (see text) are placed, in order, from the left to the right columns. In ( a – c ), dashed lines represent the criteria to determine whether the drug is exported through the 'exit' or 'cleft'. For clarity of the figures, once a trajectory goes across the thresholds, its y axis value is frozen whereas x axis value continues to change. ( d – f ) Ternary plots of the Q scores, which show the itinerancy of the state of protomer I (see Supplementary Methods ). Only representative trajectories are drawn for clarity. Full size image Second, we tested the scenario that the protonation in the TM domain of the protomer I drives the change (the B→E type). Figure 3a shows that for all 10 trajectories the three protomers completed their structural changes successfully and the drug was exported to the exit tunnel towards the TolC channel (see also Supplementary Movie 2 ). The results are perfectly compatible with the functionally rotating mechanism and simultaneously imply that the protonation process on the B conformer drives the change of the trimer from the BEA state. In this set of simulations, after the B→E change in the protomer I (see Fig. 3d ), the next step was the conformational changes either in protomer II or III. Moreover, of eight trajectories, the drug was exported when only one or two protomers changed their conformations to the target ones (see Fig. 3a ), implying that for a successful drug export alone the completion of the overall functional rotation is not compulsory. However, the complete conformational changes in the trimer are necessary for the next cycle. The third case, the A→B type, showed that, of the 10 trajectories, only one case went right, but of 8 trajectories, the drug was exported to the cleft and of nine cases the protomer I changed from the B to the A state ( Fig. 3c and f ). Interestingly, in one exceptional case, the protomer I changed from the B to the E state and, simultaneously, the drug was exported to the exit. The current thermodynamic study suggested that, given that the BEA is the stable state with one drug bound to the B protomer, the drug dissociation stabilizes the AAA state. This needs some remarks. First, this does not mean the AAA state is the functional on-pathway state. In particular, the dynamic study under proper driving force (that is, the B→E type) did not show the AAA intermediate. Instead, it suggests that, when the medium has low concentration of AcrB ligands, the AcrB trimer falls into the AAA state. Biologically, we speculate that, by taking the 'resting' AAA state, AcrB does not transport the proton and thus can avoid the energy leak. Second, some reported crystal structures took asymmetric trimer state without bound drug [14] , [15] , [16] . It was argued that those structures may not be actually 'substrate free', but may bind detergent, a known substrate of AcrB [36] . Indeed, in a recent structure of MexB, a homologue of AcrB, one detergent molecule was identified in the binding pocket [37] . In the dynamic study, the results suggested strong correlation between the conformational change of protomer I and the drug export. To understand this correlation, here we use a rather simplified argument. As in Table 1 , each state was characterized by the opening (O) or closing (X) of the four gates: 'entrance', 'cleft', 'binding pocket' and 'exit'. Suppose that initially protomer I stays in the 'B' state and so both 'entrance' and 'binding pocket' are open; thus the drug is bound in the pocket. When the protomer I is forcibly changed from the B to the E state, the entrance, the cleft and the binding pocket are all closed, but the exit gate opens, resulting for the drug to be exported through the exit. Nevertheless, when other protomers are forced to change, in the E→A and the A→B types, almost always the protomer I jumps to the A state because the B and A states are intrinsically close to each other. This transition to the A state in the protomer I implies that both the binding pocket and the exit are closed, but the entrance and the cleft remain opened, which leads the drug to be exported through the cleft. Table 1 Structural characteristics of the three states. Full size table These results are consistent with the model recently postulated by Pos based on the analogy to the 'binding change mechanism' of F o F 1 -ATP synthase [38] . We map the drug export process of AcrB onto the ATP synthesis mode of F 1 -ATPase. For the latter, the energetic bottleneck is the dissociation of ATP, for which the mechanical work in the rotation of the central stalk is used. In AcrB, the current work showed that the drug dissociation needs to be driven for the successful functional rotation. Although it is not a priori sure to what extent the analogy to F 1 -ATPase holds for AcrB, the current simulations strongly support the analogy. Next, we discuss the drug passage routes observed in the simulations. Figures 4a and b illustrate the drug export to the exit tunnel. This exit is connected to the TolC channel and thus naturally it is the right pathway to go out from the binding pocket to the cell exterior. Figures 4c and d show the drug export to the cleft tunnel. This pathway from the binding pocket to the cleft is very clear in the crystal structure. Is this cleft tunnel a potential drug import pathway? We note that this cleft tunnel is connected to the periplasm, 15 Å apart from the membrane surface. Biologically, AcrB is supposed to grab a drug molecule from the inner membrane surface, and for this purpose, the cleft tunnel is not useful. Interestingly, Pos proposed a possible role for the cleft tunnel ('tunnel 2'), being as an alternative 'exit' for the release of non-substrates taken by accident into the binding pocket [38] . Our observations may support this idea. 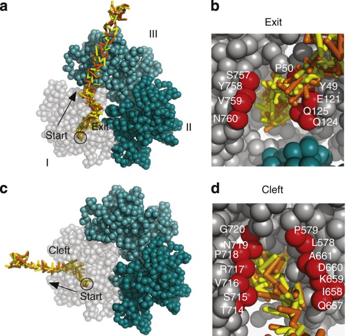Figure 4: Snapshots of drug export through 'exit' and 'cleft'. The snapshots of the drug in an exporting process are superimposed, and the odd and even time slices are in yellow and orange respectively. The protomer I is drawn transparent. The circle and arrow indicate the starting point and the direction of export respectively. (a) The drug was exported through 'exit'. (b) Closed-up view of the 'exit'; some residues are labelled and drawn in red. (c) and (d) show the drug export through the 'cleft' and the closed-up view of the 'cleft' respectively. Figure 4: Snapshots of drug export through 'exit' and 'cleft'. The snapshots of the drug in an exporting process are superimposed, and the odd and even time slices are in yellow and orange respectively. The protomer I is drawn transparent. The circle and arrow indicate the starting point and the direction of export respectively. ( a ) The drug was exported through 'exit'. ( b ) Closed-up view of the 'exit'; some residues are labelled and drawn in red. ( c ) and ( d ) show the drug export through the 'cleft' and the closed-up view of the 'cleft' respectively. Full size image Once we have the phase diagram ( Fig. 2a ), deduction to a simpler statistical model as in the reference [39] may have some merit. Indeed, we could reproduce rough, but not complete, feature of the phase diagram by calibrating parameters in the simpler model (see Methods and Supplementary Fig. S6 ). Finally, all the simulations here included the porter domain alone. The inter-domain coupling between the TM domain and the porter domain in one protomer is of essential importance, too. Reference structures The crystal structure with the PDB entry 2DRD [14] was adopted as the reference for models of both the protein, AcrB, and the drug, minocycline. In this work, three constructs were used: (1) the single protomer of the AcrB porter domain that contains L30-A183, G271-F332, P565-Q726 and E810-A873; (2) the trimer complex of the AcrB porter domain that contains the same residues as 1; (3) the trimer complex of the AcrB porter domain and some capping residues and the minocycline. The capping residues, M184-W187, A753-M781 and A215′-A236′, belonging to the TolC docking domain participate to the exit tunnel, where the prime means the residue belonging to the neighbouring protomer (see Supplementary Fig. S4 ). The symmetric structure with the PDB entry 1IWG [13] was also considered merely for a comparison with 2DRD. All the structural graphics were drawn by PyMOL ( http://www.pymol.org ). Coarse-grained model We briefly summarize the simulation model and the details are found in the Supplementary Methods . The protein was simplified by using one bead, placed on the position of C α atom, per one amino acid. For each porter domain of the protomer, the multiple-basin model [25] with three basins was used, where the three fiducial structures correspond to the B, E and A structures of 2DRD. Because the inter-protomer interactions are crucial for the allosteric effect, we treated them with much caution. We modelled them using the asymmetric AcrB structure, 2DRD, which has the three inter-protomer interfaces: for the pairs that are in contacts in all the three interfaces (the com3 set), we used a triple-well pairwise potential somewhat similar to used in refs [40] , [41] . In a similar way, the com2 pairs were modelled by a double-well pairwise potential, and the spec pairs were modelled by the Lennard-Jones-type potential (see Supplementary Fig. S5 ). To determine the relative depths of the wells for these inter-protomer interactions, we estimated the residue–residue pairwise energies of the corresponding pair at the asymmetric structure using the all-atom energy function, AMBER (version 10) ff99sb force field [42] , [43] with a GB/SA implicit solvent model [44] , [45] . We found that the com3 pairs, on average, have the strongest attraction, and the spec pairs have the weakest attraction, which was used to determine the relative depths of the wells. The minocycline, drug, was represented by six beads connected by pseudobonds between neighbours and placed at the positions of carbon atoms (in a bonded order) C21, C20, C17, C8, C13 and C71. The molecule was modelled as essentially rigid. Interactions between the drug and AcrB consist of two terms: (1) a generic repulsive term for all the pairs, and (2) the hydrophobic attraction similar to that used in ref. 27 between the drug beads and the residues in the binding pocket of AcrB, A47, Y49, P50, L177, F178, Y275, I277, I278, A279, A286, L289, F610, A611, V612, F615 and I626. Simulation protocols All the CG simulations were performed by the CafeMol package ( http://www.cafemol.org ). We conducted three sets of simulations: (1) for single-protomer simulations, 20 independent trajectories were run, each with 1.2×10 6 steps for the equilibration and 1.9×10 7 steps for the production. (2) For the trimer equilibrium simulations, 100 independent trajectories were run, each having 2.0×10 6 steps for the equilibration and 1.9×10 7 steps for the production. (3) In the simulation of drug export dynamics, 10 trajectories were run for each type of 'driving force' (see above). Each trajectory has 2.0×10 5 steps before the switching of energy landscape and 6.0×10 6 steps afterwards. All the CG simulations were carried out in constant temperature with Berendsen's thermostat [46] at the temperature T =0.24 (the Boltzmann constant k B was set to 1 in the current unit of temperature). The state of the protomer was monitored by the fraction of formation of certain native contacts, called Q score. To monitor the closeness to the E state, for example, we used a set of residue pairs that are in contact in the E state, but not in contact in the B or the A state. These 'E-specific' contacts monitor the closeness to the E state (see Supplementary Methods for more details). Statistical model A simple statistical model, similar to that used in the previous work [39] , was built to compare with the current CG model. Each protomer takes one of the three states, A, B and E, and the trimer state defined by the triplet of states has the effective energy, where the intra-energy of the protomer i , V i , takes one of the three state energies, Δ V A (=0), Δ V B and Δ V E , which correspond to the δ B and δ E respectively, in Figure 2a, and U i/j is the interaction energy between protomers, i and j . The thermodynamic probability of the trimer state is written by, as usual, p =exp(− V / T )/∑ exp(− V / T ), where the sum takes over all the trimer states. The interaction energy, Δ U ij , was initially estimated by the average energy of interface derived from the CG simulation (see Supplementary Fig. S1 ), and then they were calibrated to generate a phase diagram similar to that obtained by the simulation (see Supplementary Fig. S6 ). How to cite this article: Yao, X.-Q. et al . Drug export and allosteric coupling in a multidrug transporter revealed by molecular simulations. Nat. Commun. 1:117 doi: 10.1038/ncomms1116 (2010).